GAS2encodes a 2-oxoglutarate dependent dioxygenase involved in ABA catabolism 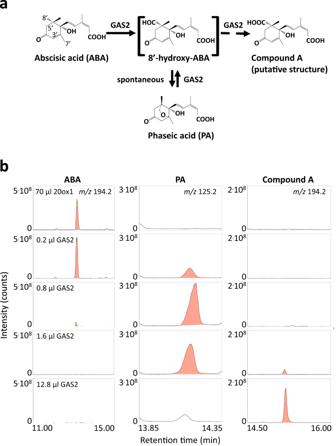Fig. 1: GAS2 is an ABA catabolising oxidase. aThe proposed ABA catabolic pathway catalysed by GAS2.bMetabolism of 3’,5’,5’,7’,7’,7’-d6-ABA incubated with 70 µL cell lysate containing recombinant ATGA20ox1 and cofactors (negative control, top lane). Metabolism ofd6-ABA incubated with indicated volumes of cell lysates containing recombinant GAS2 and cofactors as described in Methods. Chromatograms of characteristic single ions are shown in the first row for ABA (extracted ionm/z194.2), in the middle row for PA (m/z125.2), and in the right row for compound A (m/z194.2). Compounds that were identified on the basis of their full scan mass spectra of the methyl ester derivatives are shown in red. Similar results were obtained with two recombinant GAS2 preparations, produced from independent isolatedE.coliclones, each were incubated at seven different lysate concentrations. Heterologous expression of recombinant GAS2 and GA20ox1 At GAS2 (AT2G36690) and AtGA20ox1 (AT4G25420) coding sequences were custom synthesised in the pET21a expression vector (BioCat), and sequence identities were verified by sequencing on both strands. The respective plasmid DNAs were used to transform BL21 Star TM E. coli (Invitrogen) according to the manufacturer’s instructions. From the transformation reaction, 200 µL were used to inoculate 10 mL L-broth medium supplemented with carbenicillin (50 µg·mL −1 ), and transformed E. coli were grown for 16 h at 37 °C with shaking (250 rpm). From the previous E. coli culture, 2 mL were grown shaking (250 rpm) at 30 °C in 100 mL 2× YT broth with carbenicillin to OD 600 between 0.7 and 1. Expression was induced by the addition of IPTG to 1 mM; the culture was grown for a further 2 h at 30 °C and harvested by centrifugation (5,000 × g for 10 min at 4 °C). The pellet was resuspended in 200 µL of 200 mM Tris, pH 7.8 at 4 °C, containing 10 mM DTT and 1 mg . mL −1 lysozyme and the cells were disrupted by incubating on ice for 30 min, followed by four cycles of freezing in liquid N 2 and thawing. DNaseI (20U in 10 µL) were added to the E. coli cell lysate and incubated for 15 min at 20 °C. The lysates were centrifuged at 30,000 × g for 30 min at 4 °C to give approximately 500 µL of supernatant, which was used for enzyme assays [8] , [9] . Enzyme assays and purification of incubation products 3′,5′,5′,7′,7′,7′- d 6 -labelled ABA was purchased from OlChemIm, Czech Republic. PA and 7′,7′,7′- d3 -PA were gifts from Professor Eiji Nambara (University of Toronto, Canada). Preparations of E. coli cell lysates were incubated in a total volume of 100 µL containing 100 mM Tris-HCl, pH 7.0 at 30 °C for 16 h with 2-oxoglutarate and ascorbate (100 mM each, final concentrations), FeSO 4 (0.5 mM), catalase (1 mg·mL −1 ), and the substrates (5 µL in methanol) ABA (500 ng), 3′,5′,5′,7′,7′,7′- d 6 -labelled ABA (500 ng), PA (500 ng), or 7′,7′,7′- d3 -labelled PA (50 ng). Variations to the standard incubation conditions are indicated in the individual experiments. The enzymatic reactions were stopped by adding 10 µL acetic acid, which lowered the pH to about 3.2 and the incubation products were extracted two times with 500 µL methanol. The methanolic extracts were diluted with water (10 mL), containing 1% (v/v) acetic acid. The samples were loaded onto a C 18 reverse-phase Sep-Pak cartridge (Waters) and the cartridge was washed with water (2 × 10 mL), containing 1% (v/v) acetic acid. ABA incubation products were eluted from the cartridge with 80% (v/v) methanol-water, containing 1% (v/v) acetic acid. The eluates were dried under N 2 and redissolved in 200 µL methanol-water, containing 1% acetic acid (1:1), and applied to a C 18 reverse-phase column (10 cm long, 8 mm i.d., 4 mm particle size, Nova-Pak liquid chromatography cartridge in a RCM100 radial compression system; Waters), which was eluted using gradients of increasing methanol in water, containing 1% acetic acid, at 1 mL . min −1 as follows: 50% methanol, followed by five 0.5-min steps to 57.4%, 60.6%, 61.8%, 62.3%, 62.5%, one 5-min step to 62.7%, one 1-min step to 63.2% and seven 2-min steps to 64.3%, 67.2%, 70.5%, 74.9%, 81%, 89% and 100% methanol [13] . PA and compound A eluted between 3 and 6 min, and ABA between 6 and 9 min. The dried HPLC-fractions were redissolved in 100 µL methanol and methylated with 100 µL ethereal diazomethane. Samples were then transferred to glass ampoules, dried, and redissolved in 2–4 µL dichloromethane and subjected to full-scan GC-MS analysis (see below). GC-MS analysis The derivatized samples were analysed using a Thermo Scientific MS system ISQ 7000 with Advanced Electron Ionization (AEI) source equipped with a Thermo Scientific Trace 1300 gas chromatograph (GC-MS). The performance of the GC-MS was evaluated every day prior analyses by injecting authentic GA 4 as Me ester TMSi ether (0.1 ng in 1 µL in MSTFA). Samples (1–2 µL) were injected into an Agilent DB-5MS UI capillary column (30 m long, 0.25 mm i.d., 0.25 µm film thickness; Agilent, USA) at an oven temperature of 60 °C. The split value (30:1) was opened after 1 min, after which the temperature was increased by 45 °C min −1 to 175 °C and then with 4 °C min −1 to 280 °C. The He inlet was pneumatic pressure controlled at a constant flow rate of 1.2 mL . min −1 , and the injector, transfer line, and source temperatures were 280 °C, 280 °C and 250 °C, respectively. Mass spectra were acquired from 5 to 30 min after injection at an electron energy of 45 eV from 60 to 660 atomic mass units at 0.2 s per scan. For determination of Kovats retention index (KRI), 0.5 µL solution of 1 cm 2 parafilm in 2 mL hexane was injected. Reporting summary Further information on research design is available in the Nature Portfolio Reporting Summary linked to this article.